One-piece micropumps from liquid crystalline core-shell particles Responsive polymers are low-cost, light weight and flexible, and thus an attractive class of materials for the integration into micromechanical and lab-on-chip systems. Triggered by external stimuli, liquid crystalline elastomers are able to perform mechanical motion and can be utilized as microactuators. Here we present the fabrication of one-piece micropumps from liquid crystalline core-shell elastomer particles via a microfluidic double-emulsion process, the continuous nature of which enables a low-cost and rapid production. The liquid crystalline elastomer shell contains a liquid core, which is reversibly pumped into and out of the particle by actuation of the liquid crystalline shell in a jellyfish-like motion. The liquid crystalline elastomer shells have the potential to be integrated into a microfluidic system as micropumps that do not require additional components, except passive channel connectors and a trigger for actuation. This renders elaborate and high-cost micromachining techniques, which are otherwise required for obtaining microstructures with pump function, unnecessary. Microelectromechanical systems already form an integral part in our everyday lives, may it be as accelerometers for airbag deployment in cars, piezoelectrics in thermal drop-on-demand inkjet printers or biosensors in medical applications [1] , [2] . This demonstrates the need for miniature-sized mechanical actuators. From day one, it has however been a challenge to manufacture microelectromechanical systems and other types of micromechanical actuator systems with a specific shape. Lithographic methods, etching processes and specially designed micromachines have been employed for their fabrication. Therefore, silicones, shape-memory alloys and piezoceramics have been the most widely used materials [3] , [4] . In recent years, shape-memory polymers have attracted considerable interest as active materials for responsive devices [5] . They are cheap, ecologically compatible and—due to their elasticity—fracture resistant, to name only a few key advantages for a potential use as actuators. In particular, liquid crystalline elastomers (LCEs) uniquely combine the elasticity of elastomers with the anisotropic self-organization of liquid crystals as a basis for mechanical actuation [6] , [7] , [8] , [9] , [10] , [11] , [12] . The microscopic transition from the ordered but soft mesophase to the isotropic state can be triggered by temperature, light or electric fields [13] , and results in a directed macroscopic change of shape that can reach up to 400%, matching the performance of skeletal muscles [14] , [15] . Crucial to the preparation of LCEs is the uniform orientation of the anisotropic structural units, the so-called mesogens, along a common axis, the director. Commonly done in a two-step crosslinking process accompanied by mechanical stretching of a film [16] , novel approaches such as micro- and nano-templating [17] , [18] and inkjet printing techniques [19] recently opened up new possibilities to downscale LCE actuators for micro-sized applications. Ohm et al . [20] , [21] designed a microfluidic set-up that allows a continuous production of micrometre-sized LCE fibres and particles by photopolymerization of an LC monomer to obtain LCEs with customizable actuator geometry and control over the orientation of the director. Although the actuating properties of LCEs have mainly been exploited to simply trigger motion, more sophisticated applications such as peristaltic pumps and self-propelled robots have been proposed theoretically [22] . So far, a millimetre-sized motor propelled by photo-induced deformations of an LCE film and a microvalve for microfluidics with an actuating LCE film could be realized [23] , [24] . Besides microvalves, diaphragm and peristaltic micropumps are crucial for flow regulation in microchannels, which are commonly used in lab-on-chip systems. Micromechanical systems are typically prepared by microfabricating procedures, with the drawback of having to be performed in a clean room at high cost. In that respect, soft lithographic methods have easier process parameters, but to achieve a three-dimensional active device from the two-dimensional patterned elastomer layers, multi-layer structures have to be assembled. On the basis of this principle, a peristaltic micropump could be realized via a series of replica moulding from multiple templates [25] . In this contribution, we present the successful continuous fabrication of one-piece micropumps from a thermo-responsive LCE, which requires no elaborate micromachining techniques. They have the potential for further incorporation into three-dimensional microfluidic systems, whereas present-day valveless lab-on-chip micropumps, commonly made of poly(dimethylsiloxane), are generally restricted to two-dimensional flow. Preparation of core-shell elastomers in a microfluidic set-up Inspired by the contraction–pulsation movement of a jellyfish, we aimed to create an analogous synthetic microsystem: one muscle-like shell, which reversibly contracts to push and pull a liquid core into and out of the shell. For this purpose, shape-changing LCE shells filled with a liquid core were produced for the first time in a specially designed microfluidic set-up, depicted in Fig. 1a . It allows for a facile and continuous fabrication of core-shell particles with controlled size. In our system no surfactants or shell stabilizers were introduced, as they might have influenced the LC orientation [26] , which is the essential factor determining the actuation effect. The co-flow microfluidic geometry was specially chosen, as it allowed a good control of the preparation of core-shell particles [27] , [28] , and as coalescence of the particles can be avoided until they are photo-polymerized further downstream. The microfluidic device comprised a triple co-flow channel; a cylindrical glass micropipette was nested into a tapered square glass capillary, which was confined by teflon tubing. The combination of concentric cylindrical and square cross-section geometries allowed one fluid (the middle phase: the LC monomer) to flow in the voids between the circular and square capillaries, and another fluid (the inner phase: glycerol) to flow through the innermost circular channel. In Fig. 1 the inner and middle phases are drawn orange and blue, respectively. Droplets of glycerol form at the inner capillary tip and detach into the co-flowing monomer phase delivered through the square capillary. The monomer phase was designed immiscible with the other fluids, including the outer phase (silicone oil; drawn yellow), which flows in the outer-most teflon tube. This resulted in glycerol droplets encapsulated by a monomer shell that were suspended in the continuous-phase silicone oil. 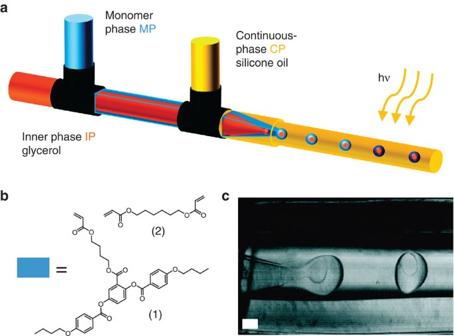Figure 1: Preparation of the core-shell elastomers. (a) The triple co-flowing geometry of the microfluidic set-up allows the fabrication of nematic shell particles filled with a glycerol core. Dispersed in the surrounding continuous-phase silicone oil, the monomer droplets are polymerized by ultraviolet light. (b) Chemical structures of the reactive mesogen (1) and crosslinker (2) in the monomer mixture. (c) Core-shell droplet formation at the capillary tip (scale bar, 100 μm). Figure 1: Preparation of the core-shell elastomers. ( a ) The triple co-flowing geometry of the microfluidic set-up allows the fabrication of nematic shell particles filled with a glycerol core. Dispersed in the surrounding continuous-phase silicone oil, the monomer droplets are polymerized by ultraviolet light. ( b ) Chemical structures of the reactive mesogen (1) and crosslinker (2) in the monomer mixture. ( c ) Core-shell droplet formation at the capillary tip (scale bar, 100 μm). Full size image Following previously derived relations between the LCE droplet size, flow rates and actuation properties [29] , we chose glass capillary tips with an orifice diameter of 20 μm for the inner cylindrical capillary and 100 μm for the square capillary to provide for a well-oriented LCE shell, which is the pre-condition for large actuation response. We decided on using glycerol for the inner phase and, hence, as the core of the core-shell particles. Glycerol is immiscible with the monomer phase and exhibits a sufficiently low viscosity at elevated temperatures (see Supplementary Table S1 ). It may be seen as a model fluid in the interior of the micropump, but it is interchangeable with other liquids after the fabrication of the latter. The LCE shell composed the three-core mesogen shown in Fig. 1b , which has previously been processed in microfluidic and templating devices [17] , [18] , [30] , but not for making core-shell particles. Attached to the rigid mesogenic unit are three flexible side chains, one of which comprises a polymerizable acrylate group. The monomer exhibits a nematic phase between 72 °C and 98 °C [15] . By addition of the non-mesogenic photoinitiator (3 wt% Lucirin TPO) and crosslinker (10 mol% 1,6-hexanedioldiacrylate), a crystalline-isotropic phase transition is observed on heating (80 °C), without any intermediate liquid crystalline regime. However, a supercooled nematic phase forms below the melting point at 80 °C on cooling. This monotropic LC phase is of sufficient stability for our LCE-shell production purposes. The low viscosity of the monomer in its high-temperature isotropic phase makes it easily processable in a microfluidic device (formation of the core-shell particles), whereas the monotropic nematic state formed at lower temperatures within the polymerization tube allows flow-induced orientation and photopolymerization to prepare oriented LCEs. Previous work on LC shells was limited to low-molecular weight, non-polymerizable mesogens, which exhibit isotropization temperatures slightly above room temperature. They could thus be manufactured at moderate temperatures in a surrounding aqueous medium [31] , [32] , [33] , [34] . With an isotropization temperature of 80 °C, the reactive monomer mixture used in this study needs to be processed at elevated temperatures and requires a customized heat-resistant microfluidic device [30] . Thus, temperature-tolerant silicone oil was chosen as the outer continuous phase. Precise control over temperature is enabled by mounting the microfluidic set-up on two hot stages: the core-shell droplets are formed at the capillary tip in the isotropic phase at 90 °C, whereas the polymerization tube is set to 65 °C, well within the nematic phase of the monomer mixture. The flow-induced orientation of the mesogens is permanently fixed through ultraviolet-initiated polymerization and crosslinking. At flow rates of 1.7 ml h −1 for the continuous phase, 0.06 ml h −1 for the monomer phase and 0.01 ml h −1 for the inner phase, about 100 core-shell elastomers are obtained per minute, dispersed in silicone oil. This allows them to be easily collected in a vessel. Characterization of the core-shell elastomers After the ultraviolet-induced polymerization, the particles consist of a cross-linked LC elastomer shell formed after full conversion of the LC monomer and crosslinker [29] . For swelling ratios see [29] and for the Young’s modulus of a comparable film (0.4 MPa) see ref. 15 . They were characterized by light microscopy, some example images are shown in Fig. 2a . At room temperature, the ellipsoidal-shaped particles possess a minimum aspect ratio (length a/width b) of 1.3. The average length of the main axis a is 545 μm with a size dispersity below 2%. The particles can be flipped manually around their main axis to reveal a third axis c, which is slightly shorter than b ( Fig. 2b ). The aspect ratio between a and c is 1.5. 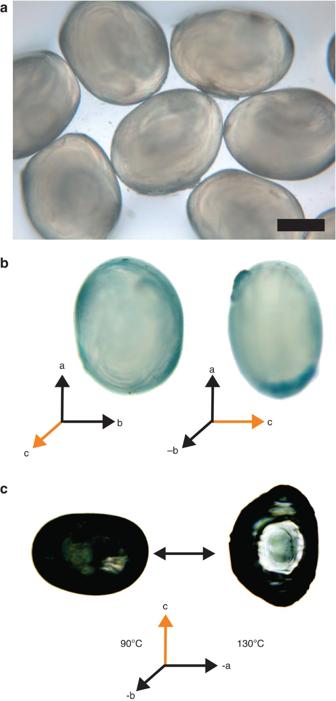Figure 2: Characterization of the core-shell elastomer particles by light microscopy. (a) Examples of the ellipsoidal-shaped core-shell particles at room temperature. (b) Top view of a particle at room temperature (on the left) and the same particle flipped around its longest axis a, revealing a shorter axis c (on the right). (c) Heating experiment demonstrating the actuation behaviour at the nematic—isotropic phase transition. The particle elongates along its short axis c. Note the glycerol core becoming visible above the clearing temperature (scale bar, 200 μm). Figure 2c shows a core-shell elastomer particle with its main axis in the horizontal and its smallest axis in the vertical direction in the nematic phase at 90 °C. In this context it should be noted that the polymerization of the monomer to an LCE increases the phase-transition temperature (nematic–isotropic) from 80 °C (monomer mixture) to 130 °C. Upon heating to the isotropic state at 130 °C, the particle shrinks along its original main axis a and expands along its initially shortest axis c. This is comparable to the behaviour of bulk particles from LCEs [20] , [29] . The aspect ratio changes from 1.5 at room temperature to 0.73 at 130 °C. The relative length change, defined as the ratio between the axis c in the actuated state and at room temperature, is 1.52. This reversible shape change leaves the total volume of the particle shell and core constant, as the core and shell have low compressibilities and the density of the nematic and isotropic phase is rather similar. This does, however, not imply that there is no hydrostatic pressure build-up. Figure 2: Characterization of the core-shell elastomer particles by light microscopy. ( a ) Examples of the ellipsoidal-shaped core-shell particles at room temperature. ( b ) Top view of a particle at room temperature (on the left) and the same particle flipped around its longest axis a, revealing a shorter axis c (on the right). ( c ) Heating experiment demonstrating the actuation behaviour at the nematic—isotropic phase transition. The particle elongates along its short axis c. Note the glycerol core becoming visible above the clearing temperature (scale bar, 200 μm). Full size image Core-shell elastomers as active micropumps To verify the concept of a micropump for our core-shell elastomers, we developed a set-up in which we could puncture the shell of the LCE to create an outlet for the glycerol core, and also easily heat the particle to the isotropic phase. A schematic drawing of the micromanipulator is shown in Fig. 3a . A glass capillary with an orifice of 40 μm in diameter and a cone angle of 3° for the capillary tip was clamped into an axially translatable holder. The core-shell particle was mounted on a glass slide between a hot plate and the capillary tip. As glycerol is very polar and exhibits an affinity for glass, the surface of the glass capillary was hydrophobized with trichloro(3,3,3-trifluoropropyl)silane to suppress potential wetting. For a better handling, the particle was heated to 90 °C, which is well above its glass-transition temperature, and pierced with the capillary tip in the rubbery state. As soon as the capillary penetrated the shell, a fraction of the liquid glycerol core rose into the capillary, due to the pressure on the pinched particle ( Fig. 3b ). Once the particle was lifted away from the hot plate, almost all liquid sank back into the particle core. 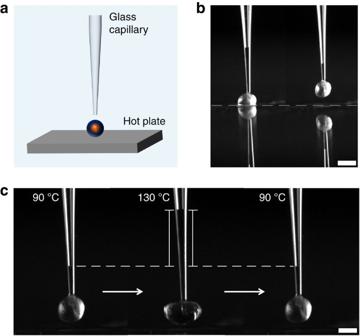Figure 3: Core-shell elastomer particles as micropumps. (a) Schematic drawing of the micromanipulator to penetrate the particle shell with a thin glass capillary. (b) Piercing the particle at 90 °C (above its glass-transition temperature) squeezes the particle between hot plate and capillary, and results in glycerol rising into the capillary. Most liquid sinks back into the core once it is lifted off the hot plate (scale bar, 100 μm). (c) When heated to the isotropic phase at 130 °C, the phase transition results in a deformation of the LCE shell. The force exerted by the actuating shell pushes the liquid glycerol core into the capillary. Once the particle resumes its former shape in the nematic phase at 90 °C, the glycerol sinks to its original level (scale bar, 100 μm). Figure 3: Core-shell elastomer particles as micropumps. ( a ) Schematic drawing of the micromanipulator to penetrate the particle shell with a thin glass capillary. ( b ) Piercing the particle at 90 °C (above its glass-transition temperature) squeezes the particle between hot plate and capillary, and results in glycerol rising into the capillary. Most liquid sinks back into the core once it is lifted off the hot plate (scale bar, 100 μm). ( c ) When heated to the isotropic phase at 130 °C, the phase transition results in a deformation of the LCE shell. The force exerted by the actuating shell pushes the liquid glycerol core into the capillary. Once the particle resumes its former shape in the nematic phase at 90 °C, the glycerol sinks to its original level (scale bar, 100 μm). Full size image The hot plate was then set to heat from 90 °C to 130 °C, which corresponds to the liquid crystalline-isotropic transition temperature of the elastomer, and the core-shell particle was slowly lowered towards the hot plate. The emitted heat induced the phase transition from nematic to isotropic within the shell, causing the particle to actuate a few millimetres away from the surface of the hot plate. At 130 °C, the punctured LC core-shell elastomer reached the isotropic phase and consequently changed its shape, in analogy to the non-punctured particles ( Fig. 2 ), but now at a constant hydrostatic pressure of the glycerol core. The shape deformation is then coupled to a corresponding reduction in core volume, leading to the expulsion of a considerable fraction of the glycerol through the shell hole and thus raising the liquid level in the capillary ( Fig. 3c ). Upon cooling, the particle reverts back to its original shape, causing the level of glycerol in the capillary to drop as the liquid is again sucked into the shell. Repeated heating and cooling cycles confirm a completely reversible actuation process through a constant increase and decrease of the glycerol level in the capillary, which is directly correlated with the shape change of the elastomer shell. Supplementary Movie 1 features several heating and cooling cycles of the punctured core-shell elastomer. The actuation response time (defined as the time from 10% to 90% of the final response) of the core-shell elastomer is about 0.1 s when using a heating gun as a fast heating device ( Fig. 4 ). Upon cooling, the corresponding relaxation time is about 0.35 s, but the increase here may be due primarily to the lack of active cooling. Using simple geometric models, we estimated the relative fraction of glycerol that is expelled from the core during heating. Taking 220 μm as the average diameter of the core, as measured from the optical microscopy images in the isotropic state, and considering the amount of glycerol in the conical tip, the total volume of glycerol amounts to approximately 5.57 nl. Upon actuation of the LCE shell, the meniscus in the capillary rises 740 μm, corresponding to a volumetric change of 3.20 nl. Hence, 64% of the liquid interior is pumped out of and into the LCE shell during one actuation cycle. In comparison, the thermal expansion of glycerol only accounts for a volumetric increase of 0.35 nl. The volume pumped out as a result of the shell actuation is thus at least 2.85 nl. 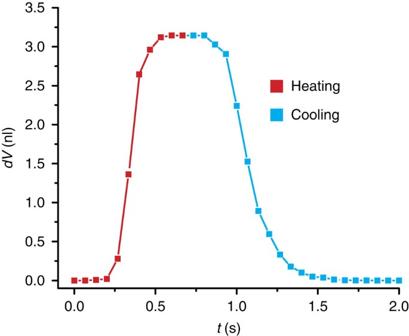Figure 4: Response speed of the micropumps upon fast heating and cooling. Heating the particle with a heat gun allows the temperature to be changed sufficiently fast to estimate the speed of actuation and relaxation (turning on and off the heat gun). The graph shows the ejected volume of glycerol as a function of time. The actuation response time is 0.1 s on heating and 0.35 s on cooling. Figure 4: Response speed of the micropumps upon fast heating and cooling. Heating the particle with a heat gun allows the temperature to be changed sufficiently fast to estimate the speed of actuation and relaxation (turning on and off the heat gun). The graph shows the ejected volume of glycerol as a function of time. The actuation response time is 0.1 s on heating and 0.35 s on cooling. Full size image Determination of the director configuration by WAXS The actuation behaviour of the elastomer particles is related to the director alignment, which can adopt several possible configurations within the nematic shell [33] . Glycerol, as well as silicone oil, promote an LC alignment with the mesogens parallel to the interface, the so-called planar alignment. Because of the interplay of LC ordering and topological confinement, the spherical topology does not allow for a defect-free planar director field [35] , and the total defect sum has to fulfil the condition s =+2 on each shell surface (internal and external). We performed wide-angle X-ray scattering (WAXS) experiments on the core-shell particles to determine the director configuration within the elastomer shell. The small diameter of the X-ray beam of only 100 μm allowed measurements of different regions within the particle ( ∼ 500 μm diameter). After a two-dimensional scan to localize the particles on the substrate, measurements were conducted at different points along the two axes a and c of the particle, as indicated in Fig. 5a . The scattering pattern of position 3 is presented in Fig. 5b . The scattering intensity profile along the scattering angle 2 θ shows two diffuse scattering maxima ( Fig. 5d ), a commonly observed motif for nematic liquid crystals. The scattering maximum at small angles corresponds to a repeat unit that reflects approximately the mesogen length, whereas the second peak in the wide-angle regime corresponds to the approximate lateral distance between the mesogens, typically 4.4 Å. 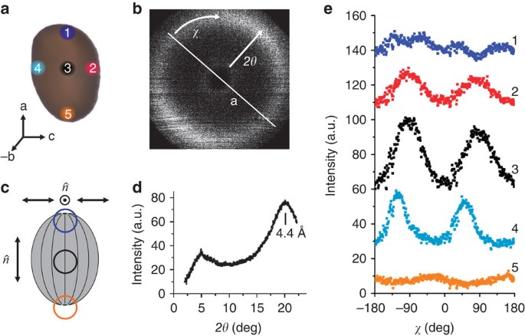Figure 5: Determination of the director configuration by WAXS. (a) Positions on the core-shell elastomer particle where the X-ray measurements were performed. (b) The scattering pattern obtained from the centre of the particle (black) as received by the detector exhibits two intensity maxima in the diffuse wide-angle signal. (c) Schematic drawing of the bipolar director alignment within the shell, depicted as seen from the outside. The approximate positions of the X-ray beam during the measurements of positions 1, 3 and 5 are highlighted. (d) The diffraction profile I(2θ) for position 3 shows two diffuse maxima at 5° and 20°, typical for nematic liquid crystals. (e) The intensities I(χ) obtained by radial integration over the wide-angle arc for positions 2, 3 and 4 exhibit two intensity maxima for nematic phases nearχ=−90° and +90°, and point to a uniform director orientation along the axis a. At the poles of the particle, the directorn^aligns normal to the axis a leading to a 90° shift of the two maxima (position 5). At position 1, the region with the director oriented parallel as well as perpendicular to the axis a is measured by the X-ray beam, leading to an intensity distribution I(χ) with four maxima. Figure 5: Determination of the director configuration by WAXS. ( a ) Positions on the core-shell elastomer particle where the X-ray measurements were performed. ( b ) The scattering pattern obtained from the centre of the particle (black) as received by the detector exhibits two intensity maxima in the diffuse wide-angle signal. ( c ) Schematic drawing of the bipolar director alignment within the shell, depicted as seen from the outside. The approximate positions of the X-ray beam during the measurements of positions 1, 3 and 5 are highlighted. ( d ) The diffraction profile I(2 θ ) for position 3 shows two diffuse maxima at 5° and 20°, typical for nematic liquid crystals. ( e ) The intensities I( χ ) obtained by radial integration over the wide-angle arc for positions 2, 3 and 4 exhibit two intensity maxima for nematic phases near χ =−90° and +90°, and point to a uniform director orientation along the axis a. At the poles of the particle, the director n^ aligns normal to the axis a leading to a 90° shift of the two maxima (position 5). At position 1, the region with the director oriented parallel as well as perpendicular to the axis a is measured by the X-ray beam, leading to an intensity distribution I( χ ) with four maxima. Full size image Information about the director orientation is provided by the azimuthal intensity distribution I( χ ) of the wide-angle halo (lateral packing). For measurements along the axis c (positions 2–4 in Fig. 5e ), radial integration over the wide-angle arc I( χ ) from 2 θ =16.0° to 22.3° yields two intensity maxima near χ =−90° and +90°, which indicates the director n^ to be aligned parallel to the main axis a [36] . In contrast, the radial intensity distributions for positions 1 and 5 near the poles of axis a exhibit intensity maxima at different angles χ . The scattering maxima of position 5 are near χ =0° and 180°, and indicate a local director field normal to the axis a. Four distinct maxima near χ =−90°, 0°, 90° and 180° observed at position 1 stem from the superposition of local preferential director orientations, both normal and parallel to the axis a. The locally resolved azimuthal intensity distribution indicates that the director is indeed aligned in a bipolar configuration along the long axis a, with point defects situated at the top and bottom of this axis ( Fig. 5c ). This director field alignment can fully explain the deformation at the phase transition presented in Fig. 2 . In such a configuration, the director n^ is preferentially oriented parallel to the axis a in most particle regions (positions 2–4), whereas around the poles the director aligns radial in all possible directions normal to the axis a (position 5). For position 1, the X-ray beam with a diameter of 100 μm samples both particle regions with director orientations perpendicular and parallel to axis a at the region vicinal to the pole. X-ray data acquired along the axes a and b of a particle flipped on its oblate side support our conclusion of a bipolar orientation and are presented in the Supplementary Figs. S1–S3 . We note that the azimuthal intensity distribution I (χ) also reflects the quality of orientational ordering and can principally be used to determine the orientational order parameter [37] , [38] . We refrain, however, from such an evaluation procedure because the scattered X-ray intensity beam does not only monitor the oriented nematic shell but also the isotropic core, the admixture of which leads to a significant underestimation of the effective order parameter. Concerning the origin of the biaxial ellipsoidal shape of the elastomers, we identified two anisotropic aspects of the LCE-shell production. First, there are two defects in the liquid crystal director fields on opposite sides of the shell, at the front and back as defined by the direction of flow and the repulsion between them can, in principle, induce an ellipsoidal shape distortion. It is, however, questionable if the forces involved are strong enough to impose any substantial distortion of the shell shape. Second, and probably more important, the absorption of optical energy during the photopolymerization is anisotropic in a fairly complex fashion. The central areas of the shell can quickly be polymerized on both sides, as the director (and thus the transition moment of the dissolved dye) is in the same plane as the polarization of the ultraviolet light, and as the thickness traversed at the top of the shell is minimal. Hence, almost the full light intensity also reaches the bottom part of the shell (here we consider the top being closest to the light source). In contrast, the peripheral regimes will be polymerized preferentially on the top side, as the light now has a much greater path through the shell, such that much light may be absorbed close to the top, leaving less intensity to polymerize the bottom. Moreover, along the shell perimeter, a considerable difference in polymerization speed can be expected between the front and back ends, on the one hand, and the intermediate region on the other. This is because the director field in the intermediate region is aligned along the flow; hence, the dye transition moment is in the same plane as the light polarization. In contrast, at the front and back, close to the director field defects, the director field is largely vertical, moving the dye transition moment out of the light polarization plane and, thus, strongly reducing the absorption cross section. Thus, the front and back ends of the shell are expected to polymerize the latest in the process. Together with the change from viscoelastic to elastic behaviour and consequent change in mechanical properties as the shell is polymerized, the time difference in polymerization at different parts of the shell may plausibly be considered to have a major role for the resulting final LCE-shell shape. The director configuration within the LC shell is a direct result from the flow profile during polymerization inside the microfluidic set-up. After detachment from the inner and middle fluid streams, the external flow of the surrounding silicone oil induces a shear flow parallel to the general flow direction at the shell exterior surface, whereas a corresponding anti-parallel shear flow must occur at the internal interface with the glycerol droplet to conserve the LC phase material. The situation is sketched in Fig. 6a for a core-shell droplet that, for simplicity, is drawn spherical. Singularities in the flow profile occur at the front and back of the shell, and these would be the natural loci of s =+1 director field defects located at each interface (internal and external). Along the shell beyond the two poles, we expect the director field to be oriented along the flow profile, as the LC normally aligns in this way to minimize flow resistance (the minimum Miesovicz viscosity η 2 is for shear flow along the director) and, thus, we would obtain a shell with bipolar director field. As the integer defects are point and not line defects, the director field within the shell is expected to ‘escape in the third dimension’ (using the terminology coined by de Gennes) along the lines connecting the inner and outer s =+1 defects at each pole. The resulting director field is sketched in Fig. 6b , as confirmed by our X-Ray measurements described above. 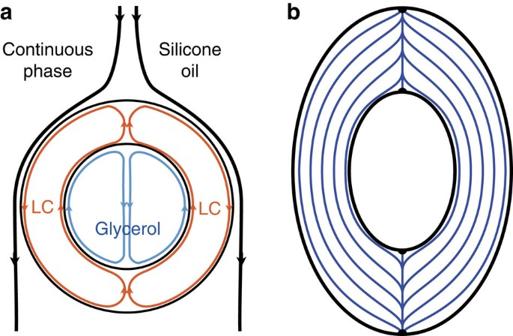Figure 6: Expected flow profile in the core-shell particles during polymerization and resulting director configuration. (a) The continuous-phase silicone oil induces a shear flow parallel to the general flow direction at the exterior surface of the shell. An anti-parallel shear flow is created at the interior interface between the monomer and glycerol. (b) Schematic drawing of the bipolar director alignment within a cross section through the middle of the shell. Singularities in the flow profile create director field defects at the internal and external interfaces. Figure 6: Expected flow profile in the core-shell particles during polymerization and resulting director configuration. ( a ) The continuous-phase silicone oil induces a shear flow parallel to the general flow direction at the exterior surface of the shell. An anti-parallel shear flow is created at the interior interface between the monomer and glycerol. ( b ) Schematic drawing of the bipolar director alignment within a cross section through the middle of the shell. Singularities in the flow profile create director field defects at the internal and external interfaces. Full size image The function of core-shell particles as micropumps is directly related to their heat-induced deformation. The change in shape happens because the nematic phase is aligned with the director along one preferred axis defined by the flow [20] , [29] , and this forces the attached polymer backbone to adopt a stretched conformation along the director, a constraint that disappears in the isotropic phase. On heating, the loss of orientational order, thus, induces a conformational change of the stretched polymer backbone to a coiled conformation [9] , [10] , [11] , [12] , [13] . For a slightly cross-linked elastomer, this microscopic transition causes a macroscopic shrinkage parallel to the director and an expansion perpendicular to it. The observed shape change of the core-shell elastomers requires a director orientation along the main axis a of the shape anisotropic (here ellipsoidal) particles as confirmed by X-ray measurements. Reciprocating micropumps rely on the periodic compression of tubes or the movement of membranes for the transport of mass. This entails the use of surrounding machinery, such as a rotor for a peristaltic pump or a reservoir for a diaphragm pump. The designed micropump from a core-shell elastomer particle here already contains an integrated reservoir and thereby reduces problems occurring in hybrid integration, for example, the glueing of components. A feasible approach to integrating our one-piece micropumps into micromechanical systems could be to employ the concept of a valveless micropump [39] , in which two anti-parallel conical diffuser/nozzle elements form the inlet and outlet of the pump. Because of their opposite geometries, they act as flow-rectifying elements and provide a one-way net fluid flow. This simple concept nicely illustrates the potential of the presented micropumps as active components on lab-on-chip devices. In conclusion, we were able, for the first time, to fabricate actuating core-shell particles from liquid crystal elastomers. Our results illustrate their potential application as micropumps and the feasibility for their integration in microelectromechanical and lab-on-chip systems. Although the presented example is limited to temperature as the response-driving external stimulus, the method of fabrication is general and can easily be adapted to different LCEs or LCE composites. By incorporating azobenzene moieties in the LCE structure, the nematic–isotropic transition can be induced by light irradiation instead of heating, thus actuating the micropump by light at a constant temperature. Alternatively, by dispersing magnetic or gold nanoparticles within the LCE material, localized inductive or plasmonic heating triggered by electromagnetic irradiation offers a different path to trigger the phase transition, and thus the actuation, even when using a temperature-responsive LCE. Using mesogens with a lower clearing temperature, a system suitable for pumping aqueous liquids would be achieved. Materials and reagents The LC side-chain monomer (4″-acryloyloxybutyl) 2,5-di(4′-butyloxybenzoyloxy)benzoate was synthesized according to literature [15] . Glycerol was obtained from Fluka. Silicone oil (1000 cSt), photoinitiator Lucirin TPO (2,4,6-trimethylbenzoyldiphenylphosphine oxide) and crosslinker 1,6-hexanedioldiacrylate were purchased from Sigma-Aldrich. The stabilizing agent was removed from 1,6-hexanedioldiacrylate by distillation. The monomer mixture used in the preparation of the core-shell particles was prepared by mixing 90 mol% monomer, 10 mol% crosslinker and 3 wt% photoinitiator in dichloromethane. Before use, the solvent was evaporated, the mixture was melted at 90 °C and drawn into a PE tube (1.78 mm inner dimension, 2.79 mm outer diameter) connected to the microfluidic channel. To obtain hydrophobic glass capillaries, the silanizing agent trichloro(3,3,3-trifluoropropyl)silane (Aldrich) was used. A stirred solution of 95 vol% ethanol/5 vol% water was adjusted to pH 4 with acetic acid and 2 wt% of the silanizing agent were added. The glass capillaries were dipped into the solution for 1 min and afterwards washed with ethanol. The coated capillaries were then cured in a vacuum oven for 1 h at 100 °C. Microfluidic device Square and round glass capillaries were purchased from Composite Metal Services (8100-100, inner dimension 1 mm) and Sutter Instrument (B100-50-10, outer diameter 1 mm), respectively. They were tapered by a micropipette puller (Sutter Instrument P97, USA) and cut to desired orifice sizes (100 μm diameter for the square and 20 μm diameter for the cylindrical capillary tip) using a microforge (Narishige MF830, Japan). The openings of the capillaries were connected to syringe pumps (Harvard 33 Double Syringe Pump) via plastic tubings. After shell formation, the droplets were polymerized by an ultraviolet lamp from LOT Oriel LSH302 (500 W), equipped with a waveguide and a 323- to 358-nm gap filter. Optical characterization of the core-shell particles The formation of the core-shell droplets in the microfluidic reactor was observed with the Zeiss stereo microscope Stemi 2000-C equipped with an Olympus XM10 camera. The heating experiments (hot-stage Linkam TMS 94) were visualized with the optical microscope Olympus BX51 equipped with the camera ColorView II. Measurement of particle size dispersity The dimensions of the core-shell particles were evaluated under the optical microscope Olympus BX51 equipped with the camera ColorView II, using the imaging software Cell^D. The ellipsoidally shaped particles had to be manually flipped on a glass slide to allow measurements of all three different axes. By default, the core-shell particles tend to lie on their flattest side. This allows the longest axes a and b to be determined, whereas axis c is oriented along the direction of view. The particle was then flipped 90° about axis a, such that axis c could be measured. Inevitably, when doing such a sensitive manipulation by hand, the tilting angle was not always precisely 90° and the particles were easily askew, leading to less accurate size determination and, consequently, slightly larger size dispersities for axes b and c than for axis a (see Supplementary Fig. S4 for bar plots). A total of 20 particles were measured, giving the following results: axis a: 545 μm (±10 μm, ±2%); axis b: 413 μm (±18 μm, ±4%); axis c: 364 μm (±12 μm, ±3%). WAXS experiments The WAXS experiments were performed with a Bruker NanoStar diffractometer, equipped with a HiStar area detector and crossed Goebel mirrors, using CuK α ( λ =1.5418 Å) radiation. How to cite this article : Fleischmann E.-K. et al . One-piece micropumps from liquid crystalline core-shell particles. Nat. Commun. 3:1178 doi: 10.1038/ncomms2193 (2012).